Changing the peptide specificity of a human T-cell receptor by directed evolution Binding of a T-cell receptor (TCR) to a peptide/major histocompatibility complex is the key interaction involved in antigen specificity of T cells. The recognition involves up to six complementarity determining regions (CDR) of the TCR. Efforts to examine the structural basis of these interactions and to exploit them in adoptive T-cell therapies has required the isolation of specific T-cell clones and their clonotypic TCRs. Here we describe a strategy using in vitro -directed evolution of a single TCR to change its peptide specificity, thereby avoiding the need to isolate T-cell clones. The human TCR A6, which recognizes the viral peptide Tax/HLA-A2, was converted to TCR variants that recognized the cancer peptide MART1/HLA-A2. Mutational studies and molecular dynamics simulations identified CDR residues that were predicted to be important in the specificity switch. Thus, in vitro engineering strategies alone can be used to discover TCRs with desired specificities. Heterodimeric αβ T-cell receptors (TCRs) are responsible for recognizing antigenic peptides presented in the context of a product of the major histocompatibility complex (MHC) on the surface of antigen-presenting cells. The interaction of a TCR and a peptide/MHC (pepMHC) can drive the T cell into various states of activation, depending on the affinity (or dissociation rate) of binding. This recognition also operates during thymic development of a T cell in a process that selects for T cells with TCRs that bind with low affinity to self-pepMHC complexes (positive selection), but deletes T cells with TCRs that bind too strongly to self-pepMHC complexes (negative selection or tolerance) [1] , [2] . T cells exported to the periphery are thus positioned to discriminate between a normal, healthy cell and one that expresses aberrant pepMHC due to an infectious agent such as a virus or due to cell transformation to a cancerous state. TCRs contain six complementarity determining regions (CDRs), three (CDR1, CDR2 and CDR3) in each α- and β-chain, which are involved in binding pepMHC ligands. Based on the solved TCR:pepMHC structures [3] , [4] , a common diagonal docking orientation positions the TCR such that the CDR1 and CDR2 loops encoded by the germline variable (V) region genes are typically positioned over the helices of the MHC. The CDR3 loops of each chain are encoded by nucleotides at the junctions of somatically rearranged gene segments, and these hypervariable regions are appropriately positioned over the peptide (reviewed in refs 3 , 4 ). Although it was originally thought that peptide specificity was determined in large part through interactions of CDR3 loops with the peptide, many studies have suggested that antigen specificity is more complex. For example, in an early study of I-E k -restricted TCRs that recognized distinct peptides, transplantation of CDR3 loops was not sufficient to confer peptide reactivity, even when the same Vα chains were used by the two TCRs [5] . Based on current thinking, specificity in the TCR:pepMHC interaction can occur through various mechanisms, including the following: (1) residues in the germline-encoded CDR1 loops that make direct contact with peptide [6] , [7] , [8] , [9] , (2) CDR1 and CDR2 contacts with MHC that yield peptide-specific interactions indirectly by altering MHC contact with the peptide [4] , [10] , (3) CDR3 loops that modulate contacts between CDR1/CDR2 residues and MHC [11] , [12] , [13] , [14] and (4) peptide influences that have an impact on MHC interactions with CDR1, CDR2, or even CDR3 residues [15] , [16] , [17] . Given the complexity of interloop interactions among CDRs, it is difficult to use computational approaches to predict the basis of peptide specificity by TCRs, let alone to design TCRs with novel specificities de novo . Directed evolution has been used to engineer TCRs with large improvements in binding affinity (or altered fine specificity [18] ), while maintaining antigen specificity [19] , [20] , [21] , [22] , [23] , [24] , [25] . These studies have frequently targeted CDR3 regions for mutagenesis to accomplish affinity maturation, but mutations in CDR1 and CDR2 loops have also yielded improvements in affinity while maintaining peptide specificity [21] , [22] , [23] , [25] , [26] . Furthermore, computational approaches have been used to guide improvements in TCR affinity, with only subtle effects on specificity [27] , [28] , [29] , [30] . Although affinity maturation of TCRs has been achieved, there have not been reports in which the specificity of a TCR has been changed to a completely different peptide using directed evolution (that is, from the cognate peptide to a non-cognate peptide). Here we describe the successful in vitro engineering of the human TCR A6 that recognizes a cognate nonameric peptide from the viral protein Tax, converting the TCR to one that specifically recognizes a non-cognate decameric peptide from the melanoma antigen MART1. The study shows that it is possible to use directed evolution and in vitro approaches to engineer TCRs with alternative specificities, opening the possibility for rapid discovery of TCRs against a large array of cancer, viral and autoimmune antigens. TCR A6 and selected HLA-A2-restricted peptides To test whether the specificity of a TCR could be converted to a different MHC-restricted peptide by directed evolution, we used the human TCR A6, which was originally raised against the HTLV-1 peptide Tax (LLFGYPVYV) [31] . A6 was chosen due to its thorough structural and biochemical characterization [8] , [15] , [16] , [32] , [33] , and its prior expression as a stable single-chain TCR (scTCR, Vβ-linker-Vα) in the yeast display system [34] . Our goal was to convert the A6 TCR from binding the cognate peptide Tax to binding cancer-associated MART1 peptides (nonamer, AAGIGILTV and an anchor-modified decamer, ELAGIGILTV), or WT1 (RMFPNAPYL) [35] , [36] , [37] . One of the advantages of the MART1 system is that MART1-specific TCRs have shown a preference for Vα2 (IMGT: TRAV 12-2) [38] , the same Vα region (that is, CDR1α and CDR2α) used by A6. In addition, the Vα2-containing MART1-specific TCR DMF5 targets MART1/HLA-A2 with a similar docking mode to the A6 TCR [7] , [30] . The MART1 peptides differ from Tax at every position, except the primary anchor near the carboxy terminus ( Fig. 1a,b ), and the WT1 peptide differs from Tax at every position, except positions 3 (F) and 8 (Y) ( Fig. 1a,c ). Notably, MART1 lacks the aromatic residues of Tax (that is, F3, Y5 and Y8) and exhibits a distinct backbone configuration. The anchor-modified MART1 decamer (ELAGIGILTV) binds with higher affinity to HLA-A2 than the nonamer (AAGIGILTV) [39] , although MART1-specific TCRs often cross-react with both ( Fig. 1b ) [40] , [41] . Hence, the anchor-modified decamer was used for all selections due to its enhanced binding to HLA-A2. In summary, both MART1 and WT1 present unique surfaces to the TCR for examining the notion of whether a single TCR can be engineered to bind a non-cognate peptide. 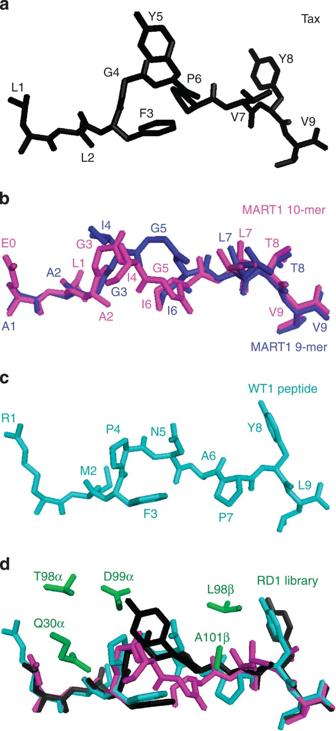Figure 1: Selecting peptide structures and RD1 library design. (a) Structure of the HLA-A2-bound Tax peptide (LLFGYPVYV)(PDB: 1DUZ)66, black. (b) Structural alignment of the HLA-A2-bound, decamer MART1 peptide (ELAGIGILTV)(PDB: 1JF1)67, magenta, and the HLA-A2-bound nonamer MART1 peptide (PDB: 2GUO)39, blue. (c) Structure of the HLA-A2-bound WT1 peptide (RMFPNAPYL)(PDB: 3HPJ)68, cyan. (d) Five residues (green), Q30α, T98α, D99α, L98β and A101β (G in the wild-type A6), generated as degenerate codons in the RD1 library, as found in the structure of the A6-c134:Tax/HLA-A2 complex (PDB: 4FTV)47. A6-c134 contains the same CDR sequences as the single-chain A6-X15 (ref.34) that was used as the RD1 library template. Tax peptide is in black, MART1 decamer peptide from the aligned Mel5:MART1/HLA-A2 structure (PDB: 3HG1)7is in magenta and WT1 peptide from the aligned WT1/HLA-A2 structure (PDB: 3HPJ)68is in cyan. Figure 1: Selecting peptide structures and RD1 library design. ( a ) Structure of the HLA-A2-bound Tax peptide (LLFGYPVYV)(PDB: 1DUZ) [66] , black. ( b ) Structural alignment of the HLA-A2-bound, decamer MART1 peptide (ELAGIGILTV)(PDB: 1JF1) [67] , magenta, and the HLA-A2-bound nonamer MART1 peptide (PDB: 2GUO) [39] , blue. ( c ) Structure of the HLA-A2-bound WT1 peptide (RMFPNAPYL)(PDB: 3HPJ) [68] , cyan. ( d ) Five residues (green), Q30α, T98α, D99α, L98β and A101β (G in the wild-type A6), generated as degenerate codons in the RD1 library, as found in the structure of the A6-c134:Tax/HLA-A2 complex (PDB: 4FTV) [47] . A6-c134 contains the same CDR sequences as the single-chain A6-X15 (ref. 34 ) that was used as the RD1 library template. Tax peptide is in black, MART1 decamer peptide from the aligned Mel5:MART1/HLA-A2 structure (PDB: 3HG1) [7] is in magenta and WT1 peptide from the aligned WT1/HLA-A2 structure (PDB: 3HPJ) [68] is in cyan. Full size image To guide the mutagenesis strategy for the construction of A6 libraries, we examined, by modelling, which residues of the A6 CDR loops would be most likely to accommodate and provide binding energy to non-cognate peptides MART1 and WT1 in the HLA-A2 complex (see Methods). Based on the results of the modelling, and on the limitations of library size in the yeast display system, we selected five CDR positions that were the most commonly represented among the complexes within this distance: TCRα Q30, T98 and D99, and TCRβ L98 and G101 (A101 in the A6-X15 template) ( Fig. 1d ) to generate the library called RD1. The RD1 library also contained four CDR3β mutations that conferred high affinity for Tax/HLA-A2 and one CDR3β mutation that conferred increased stability for yeast display ( Fig. 2 ) [34] . 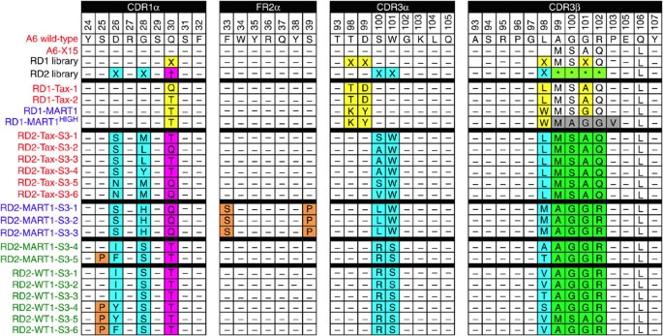Figure 2: Amino acid sequences of various A6-derived TCR clones. Residues of A6 wild-type TCR8and the high-affinity variant A6-X15 (ref.34) are shown. Positions of degeneracy in the RD1 and RD2 libraries are highlighted, where X represents any amino acid (based on NNS or NNK nucleic acid composition in yellow and cyan, respectively). RD2 position 30 indicated with ‘†’ in magenta indicates a binary position where either wild-type Q or a T was present in the library. RD2 positions 99–102 in CDR3β indicated by four consecutive ‘*’ indicate a binary string where the four adjacent residues were either A6 wild-type (AAGR) or A6-X15 (MSAQ). PCR-based mutations in selected TCR mutants are highlighted in orange. Mutants isolated from the RD1 selections are shown (RD1-Tax-1, RD1-Tax-2 and RD1-MART1) and the affinity-matured RD1-MART1 variant, RD1-MART1HIGH(selected residues from affinity maturation are highlighted in grey) as well. Sequences of other RD1 isolates are shown inSupplementary Figs 2–4. Variants selected from the RD2 library following the third sort are shown. RD2-Tax-S3-1 to S3-6 clones were specific for Tax, and RD2-MART1-S3-1 to S3-3 clones were identical and specific for MART1 (also called RD2-MART1). The RD2-MART1-S3-4 and S3-5 clones listed separately showed binding to all three peptide complexes (that is, Tax, MART1 and WT1), as did all six clones isolated with WT1/HLA-A2 (RD2-WT1-S3-1 to S3-6). Residue numbering is consistent with the crystal structures of A6:Tax/HLA-A2 (PDB: 1AO7)8and A6-c134:Tax/HLA-A2 (PDB: 4FTV)47. TCR variants names are coloured according to their determined specificities: Tax/HLA-A2 (red), MART1/HLA-A2 (blue) and cross-reactive (green). Figure 2: Amino acid sequences of various A6-derived TCR clones. Residues of A6 wild-type TCR [8] and the high-affinity variant A6-X15 (ref. 34 ) are shown. Positions of degeneracy in the RD1 and RD2 libraries are highlighted, where X represents any amino acid (based on NNS or NNK nucleic acid composition in yellow and cyan, respectively). RD2 position 30 indicated with ‘†’ in magenta indicates a binary position where either wild-type Q or a T was present in the library. RD2 positions 99–102 in CDR3β indicated by four consecutive ‘*’ indicate a binary string where the four adjacent residues were either A6 wild-type (AAGR) or A6-X15 (MSAQ). PCR-based mutations in selected TCR mutants are highlighted in orange. Mutants isolated from the RD1 selections are shown (RD1-Tax-1, RD1-Tax-2 and RD1-MART1) and the affinity-matured RD1-MART1 variant, RD1-MART1 HIGH (selected residues from affinity maturation are highlighted in grey) as well. Sequences of other RD1 isolates are shown in Supplementary Figs 2–4 . Variants selected from the RD2 library following the third sort are shown. RD2-Tax-S3-1 to S3-6 clones were specific for Tax, and RD2-MART1-S3-1 to S3-3 clones were identical and specific for MART1 (also called RD2-MART1). The RD2-MART1-S3-4 and S3-5 clones listed separately showed binding to all three peptide complexes (that is, Tax, MART1 and WT1), as did all six clones isolated with WT1/HLA-A2 (RD2-WT1-S3-1 to S3-6). Residue numbering is consistent with the crystal structures of A6:Tax/HLA-A2 (PDB: 1AO7) [8] and A6-c134:Tax/HLA-A2 (PDB: 4FTV) [47] . TCR variants names are coloured according to their determined specificities: Tax/HLA-A2 (red), MART1/HLA-A2 (blue) and cross-reactive (green). Full size image Isolation of RD1 library mutants To determine whether the RD1 library contained mutants that bound to MART1 or WT1, as well as to verify that the library contained mutants that bound to Tax, fluorescence-activated cell sorting (FACS) was used for selections with Tax/HLA-A2-Ig, MART1/HLA-A2-Ig (using the anchor-modified decamer peptide) and WT1/HLA-A2-Ig dimers. As expected, the unselected RD1 library did not show detectable positive peaks with any ligand, but a positive population began to emerge for Tax/HLA-A2 and MART1/HLA-A2 after the second and fourth sorts, respectively ( Supplementary Fig. 1a,b ). A positive peak did not emerge with WT1/HLA-A2 even after the fifth sort ( Supplementary Fig. 1c ) and thus only the Tax and MART1-reactive clones were pursued further. Two of six clones isolated from the RD1 library following sorting with Tax had identical amino acid sequences to A6-X15 (although the codons varied) and four clones had a threonine substitution at position 30 in CDR1α ( Fig. 2 and Supplementary Fig. 2 ). The similarities to A6-X15 suggest that there was strong selection for these residues in conferring high-affinity Tax binding. In addition, emergence of highly restricted residues through successive sorts also argued that the final high-affinity clones were evolved at these positions to optimize binding ( Supplementary Fig. 2 ). To determine whether the TCRs selected for binding to the Tax peptides exhibited specificity in their reaction with the selecting peptide, RD1-Tax-1 (Q30α, T98α, D99α, L98β and A101β) was titrated with various concentrations of Tax and MART1/HLA-A2-Ig dimers, at concentrations ranging from 4 to 500 nM ( Fig. 3a , top panels). The Tax-selected TCR, RD1-Tax-1, bound only to the Tax complex and not to the MART1 complex, with half-maximal binding of Tax/HLA-A2-Ig dimer at ~110 nM ( Fig. 3b ). 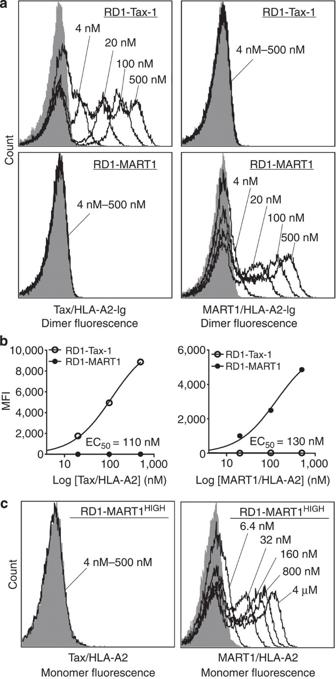Figure 3: Binding of selected RD1 TCR clones. Following four sorts of the RD1 library with Tax (LLFGYPVYV)/HLA-A2 and five sorts of the RD1 library with MART1 (ELAGIGILTV)/HLA-A2 as shown in (Supplementary Fig. 1a,b), individual yeast clones were analysed for peptide/HLA-A2 binding. (a) The RD1-Tax-1 clone isolated from Tax selections (top panels), which was identical in amino acid sequence to A6-X15, and the RD1-MART1 clone isolated from MART1 selections (bottom panels) were stained with various concentrations of the Tax/HLA-A2-Ig dimer (left panels) or MART1/HLA-A2-Ig dimer (right panels) at the indicated concentrations. Grey filled histograms were yeast cells stained with secondary antibody only. (b) Plot of the mean fluorescence intensity (MFI) from staining RD1-Tax-1 and RD1-MART1 with various concentrations of Tax/HLA-A2-Ig dimers (left) and MART1 (ELAGIGILTV)/HLA-A2-Ig dimers (right) at 4–500 nM. The half-maximal effective concentration (EC50) determined by nonlinear regression analysis is indicated. (c) The RD1-MART1HIGHclone, isolated by affinity maturation of the RD1-MART1 clone, was stained with various concentrations of Tax/HLA-A2 monomers (left panel) or MART1/HLA-A2 monomer (right panel) at the indicated concentrations. Data are representative of four experiments with similar results. Figure 3: Binding of selected RD1 TCR clones. Following four sorts of the RD1 library with Tax (LLFGYPVYV)/HLA-A2 and five sorts of the RD1 library with MART1 (ELAGIGILTV)/HLA-A2 as shown in ( Supplementary Fig. 1a,b ), individual yeast clones were analysed for peptide/HLA-A2 binding. ( a ) The RD1-Tax-1 clone isolated from Tax selections (top panels), which was identical in amino acid sequence to A6-X15, and the RD1-MART1 clone isolated from MART1 selections (bottom panels) were stained with various concentrations of the Tax/HLA-A2-Ig dimer (left panels) or MART1/HLA-A2-Ig dimer (right panels) at the indicated concentrations. Grey filled histograms were yeast cells stained with secondary antibody only. ( b ) Plot of the mean fluorescence intensity (MFI) from staining RD1-Tax-1 and RD1-MART1 with various concentrations of Tax/HLA-A2-Ig dimers (left) and MART1 (ELAGIGILTV)/HLA-A2-Ig dimers (right) at 4–500 nM. The half-maximal effective concentration (EC 50 ) determined by nonlinear regression analysis is indicated. ( c ) The RD1-MART1 HIGH clone, isolated by affinity maturation of the RD1-MART1 clone, was stained with various concentrations of Tax/HLA-A2 monomers (left panel) or MART1/HLA-A2 monomer (right panel) at the indicated concentrations. Data are representative of four experiments with similar results. Full size image Five clones isolated following the fifth sort with MART1 were sequenced and all had identical nucleotide sequences encoding T30α, K98α, Y99α, W98β and G101β (called RD1-MART1) ( Fig. 2 and Supplementary Fig. 3 ). Except for T30α and G101β, these mutations differed from the wild-type and high-affinity Tax-specific A6 scTCRs. Sequencing of clones following succesive sorts showed the emergence of selected residues (K/R) at position 98 of CDR3α during the third sort ( Supplementary Fig. 3 ). To determine whether the TCR selected for binding to MART1 exhibited specificity, the RD1-MART1 clone was titrated with various concentrations of the MART1 and Tax/HLA-A2-Ig dimers ( Fig. 3a , bottom panels). RD1-MART1 bound only to the MART1 complex, and not to the Tax complex, with half-maximal binding at ~130 nM ( Fig. 3b ). Thus, a higher-affinity TCR mutant against a distinctly different peptide could be isolated from a degenerate library of a single TCR. Affinity maturation of the MART1-selected RD1 mutant To determine whether RD1-MART1 could be engineered for even higher affinity and yet retain MART1 specificity, degenerate libraries (NNK) were made in the CDR3 loops of RD1-MART1 spanning 5-codon regions in CDR3α residues 98–102 and CDR3β residues 97–101 and 99–103 ( Supplementary Fig. 4 ). Two rounds of selection were performed with the pooled libraries, first with 200 nM MART1/HLA-A2-Ig dimers and then with 1 nM dimer, a concentration below the detectable limit for staining the parental RD1-MART1 ( Fig. 3b ). Each sort contained a positive population of yeast ( Supplementary Fig. 1d ) and ten clones from the second sort were sequenced. Eight clones contained the parental RD1-MART1 sequence, one clone contained a Q81K PCR-based mutation in the Vα region and one clone, called RD1-MART1 HIGH , had three mutations in CDR3β that differed from the parental sequence (S100A, Q102G and P103V) ( Fig. 2 and Supplementary Fig. 4 ). RD1-MART1 HIGH retained specificity for MART1 and showed significant binding with monomeric MART1/HLA-A2, whereas RD1-MART1 only showed binding at the highest monomer concentration ( Fig. 3c and Supplementary Fig. 5 ). Staining of RD1-MART1 HIGH with non-selecting cognate peptide Tax/HLA-A2 and other non-cognate peptides WT1 (RMFPNAPYL)/HLA-A2 and Survivin (LTLGEFLKL)/HLA-A2 showed no detectable signal even with 500 nM peptide/HLA-A2-Ig dimers, over 500 times the concentration of MART1/HLA-A2-Ig dimers that yielded detectable staining ( Supplementary Fig. 6 ). Design and selection of a second A6 scaffold library RD2 To determine whether alternative diversity in the A6 scaffold could be used to generate TCR mutants that are specific for MART1/HLA-A2 or WT1/HLA-A2, a second library, RD2, was designed with five degenerate (NNK) positions ( Fig. 4a ): TCRα D26, G28, S100 and W101 and TCRβ L98, a binary position at TCRα 30 (Q30 or T30) and a binary region in TCRβ 99–102 (AGGR or MSAQ) ( Fig. 2 and Methods). RD2 was screened with three pepMHC ligands, Tax/HLA-A2 (LLFGYPVYV; cognate), MART1/HLA-A2 (ELAGIGILTV; non-cognate) and WT/HLA-A2 (RMFPNAPYL; non-cognate), using two Magnetic Activated Cell Sorting (MACS) selections followed by one round of FACS. Selections with Tax, MART1 and WT1 all showed the emergence of positive populations ( Supplementary Fig. 7 ). 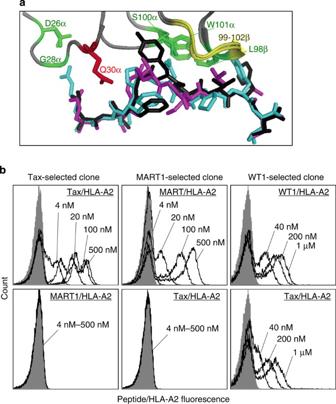Figure 4: Binding of selected RD2 TCR clones. (a) Residues of A6 TCR used in the design of the RD2 library. The structures of the aligned wild-type A6:Tax/HLA-A2 (PDB: 1AO7)8and A6-c134:Tax/HLA-A2 (PDB: 4FTV)47, which contained the CDR sequences used as templates for the RD2 library, are shown with degenerate positions at D26α, G28α, S100α, W101α and L98β (green). The binary residues (Gln or Thr) at position Q30α is shown in red and the backbone of the binary strings of wild-type ‘AGGR’ or high-affinity ‘MSAQ’ in positions 99–102β are shown in yellow. The Tax peptide is in black, the MART1 peptide from the aligned Mel5:MART1/HLA-A2 structure (PDB: 3HG1)7is in green and the WT1 peptide from the aligned WT1/HLA-A2 structure (PDB: 3HPJ)68is in cyan. (b) A Tax-selected clone (RD2-Tax-S3-1) (left panels), a MART1-selected clone (RD2-MART1) (middle panels) and a WT1-selected clone (RD2-WT1-1) were each stained with various concentrations of the indicated peptide/HLA-A2-Ig dimers. Grey filled histograms were yeast cells stained with secondary antibody only. Data are representative of three experiments with similar results. Figure 4: Binding of selected RD2 TCR clones. ( a ) Residues of A6 TCR used in the design of the RD2 library. The structures of the aligned wild-type A6:Tax/HLA-A2 (PDB: 1AO7) [8] and A6-c134:Tax/HLA-A2 (PDB: 4FTV) [47] , which contained the CDR sequences used as templates for the RD2 library, are shown with degenerate positions at D26α, G28α, S100α, W101α and L98β (green). The binary residues (Gln or Thr) at position Q30α is shown in red and the backbone of the binary strings of wild-type ‘AGGR’ or high-affinity ‘MSAQ’ in positions 99–102β are shown in yellow. The Tax peptide is in black, the MART1 peptide from the aligned Mel5:MART1/HLA-A2 structure (PDB: 3HG1) [7] is in green and the WT1 peptide from the aligned WT1/HLA-A2 structure (PDB: 3HPJ) [68] is in cyan. ( b ) A Tax-selected clone (RD2-Tax-S3-1) (left panels), a MART1-selected clone (RD2-MART1) (middle panels) and a WT1-selected clone (RD2-WT1-1) were each stained with various concentrations of the indicated peptide/HLA-A2-Ig dimers. Grey filled histograms were yeast cells stained with secondary antibody only. Data are representative of three experiments with similar results. Full size image Following selection with Tax/HLA-A2, six colonies were sequenced and analysed. Although all six clones bound to Tax/HLA-A2 but not to MART1/HLA-A2, clones RD2-Tax-1 and RD2-Tax-2 showed improved staining compared with the high-affinity A6-X15 TCR [34] when stained with Tax/HLA-A2-Ig dimers and monomers ( Fig. 4b , left panels and Supplementary Fig. 8 ). All six clones differed in sequence ( Fig. 2 ), but each retained CDR3β residues MSAQ at TCRβ positions 99–102 (rather than the wild-type binary option AGGR) that were present in the high-affinity A6-X15 TCR. Two residues that were among the positions of complete degeneracy in the library, CDR3α W101 and CDR3β L98, were also highly restricted. Thus, this constellation of residues was highly selected for binding the Tax peptide, despite the fact that the residues were present in different CDR loops. The other positions (CDR1α 26, 28, 30 and CDR3α 98) in the degenerate library were biased towards particular residues, but variability at these positions suggested that different solutions for binding Tax/HLA-A2 existed. Five clones selected with MART1/HLA-A2 all bound to MART1/HLA-A2 but three showed specificity for MART1 (that is, did not bind to Tax or WT1; Fig. 4b , centre panels), whereas the other two also bound to Tax and WT1. Sequencing revealed that the three MART1-specific clones all had the same sequence (clones RD2-MART1-S3-1, -2, -3; called RD2-MART1), whereas the two cross-reactive clones differed substantially from this sequence, but were similar to each other (clones RD2-MART1-S3-4 and -5) ( Fig. 2 ). Interestingly, unlike the Tax-selected clones, all of the MART1-selected clones contained the four CDR3β residues (AGGR) of the wild-type A6 TCR. The MART1-specific clones contained residues S26, H28 and Q30 in CDR1α, residues L100 and W101 in CDR3α and residue M98 in CDR3β. Each of these selected residues was distinctly different from the Tax-specific clones, except for the tryptophan in CDR3α (W101). This finding supports the view that all of these residues contributed either directly or indirectly to the peptide specificity of the TCRs. The MART1-specific clones also contained two mutations, to Ser and Pro at positions 33 and 39, in framework region 2 of the Vα chain that were probably incorporated through PCR errors ( Fig. 2 ). The presence of a proline in framework regions has been observed in other TCR engineering studies [42] , [43] , [44] and may be involved in stabilizing V domains, thereby enhancing yeast surface levels. The two cross-reactive clones, RD2-MART1-S3-4 and -5, shared the same residues at CDR1α S28, CDR3α R100 and CDR3α S101, but differed at CDR1α 26, CDR1α 30 and CDR3β 98. One of the clones also contained a single-site mutation to a proline at CDR1α 25. Six clones selected with WT1/HLA-A2 bound to all three peptide ligands, WT1, Tax and MART1 ( Fig. 4b , right panels), and thus showed a binding phenotype similar to the two cross-reactive MART1-selected clones (RD2-MART1-S3-4 and -5) ( Fig. 2 ). The sequences of all six clones were unique ( Fig. 2 ), but they also shared significant similarities to the MART1-selected, cross-reactive clones. All eight cross-reactive clones contained CDR1α S28, CDR3α R100 and CDR3α S101 residues, suggesting that these were important in binding to the pep/HLA-A2 complexes regardless of the peptides. Three of the WT1-selected clones also contained the proline mutation at position 25 of CDR1α and an aromatic residue at the adjacent amino acid CDR1α 26. This pair of residues may be important in configuring the TCR to bind to the ligands, again independent of the peptide. Finally, one of the clones (RD2-WT1-S3-5) contained the CDR3β residues 99–102 (MSAQ) of the high-affinity Tax-specific TCR A6-X15, suggesting that it was not absolutely critical to have the potentially more flexible CDR3β residues of the wild-type TCR A6 to generate cross-reactivity. However, the cross-reactive clones did contain residues with smaller side chains at position 98 of CDR3β, compared with the Leu, Trp or Met found with the Tax- or MART1-specific clones. Site-directed mutagenesis of RD scaffold mutants Examination of the sequences of the isolated RD1 variants suggested that TCRβ position 98 might be important in their specificity, as all Tax-specific variants contained the wild-type Leu at CDR3 β98, whereas MART1-specific variants contained either Trp (RD1-MART1) or Met (RD2-MART1). To assess whether this residue was pivotal in the specificity switch, converting A6-X15 into a MART1-specific TCR, this position was reverted to Leu in the MART1-specific mutants (W98L for RD1-MART1 and RD1-MART1 HIGH , and M98L for RD2-MART1). Conversely, the RD1-Tax-1 clone (A6-X15) was mutated to the residues selected in the MART1-specific variants (L98W and L98M). Yeast-displayed mutants were stained with peptide/HLA-A2 tetramers ( Fig. 5 ) and the results showed that the residue selected at position 98 was critical for binding. The only exceptions were that: (1) the L98M mutation in A6-X15 resulted in binding to Tax/HLA-A2, but at a reduced level ( Fig. 5a and Supplementary Fig. 9 ), and (2) the M98L reversion mutation of RD2-MART1 maintained specific binding to MART1. In no case was the specificity of the original TCR reverted to high-affinity binding of the alternative peptide, even at concentrations of pep/HLA-A2 tetramers that were 20-fold above detectable levels with the original clone. We conclude that residues at position 98 were important for high-affinity binding and specificity (except for the RD2-MART1 clone), but this mutation alone was not responsible for the switch in peptide specificity. Interestingly, the MART1-specific TCR DMF5 has a Leu at position β98, but mutation of this position to tryptophan enhanced affinity by >3-fold [30] . Finally, Rosetta sequence tolerance algorithms were used to determine whether residues other than the wild-type leucine had a significant probability of tolerance at the A6-c134:Tax/HLA-A2 interface ( Supplementary Fig. 10a ). The results showed that leucine was by far the most tolerated amino acid (predicted frequency of 90–100%), whereas all other amino acids combined yielded a frequency of <10%. 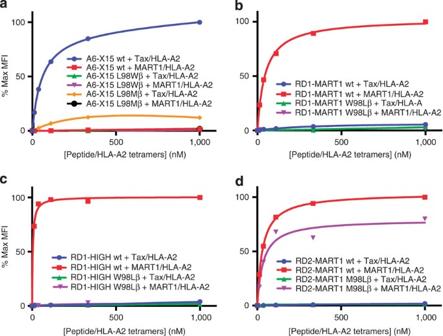Figure 5: Binding analysis of position 98β mutants of selected TCRs. Binding titrations of the indicated mutants of A6-X15 (a), RD1-MART1 (b), RD1-MART1HIGH(c) and RD2-MART1 (d). Mutants were stained with 12.3, 37.0, 111, 333, and 1000, nM Tax and MART/HLA-A2 PE-conjugated streptavidin tetramers. Normalized per cent max mean fluorescence intensity (MFI) is plotted against peptide/HLA-A2 tetramer concentration. This experiment was also performed with pepMHC-Ig dimers with similar results (Supplementary Fig. 9). Figure 5: Binding analysis of position 98β mutants of selected TCRs. Binding titrations of the indicated mutants of A6-X15 ( a ), RD1-MART1 ( b ), RD1-MART1 HIGH ( c ) and RD2-MART1 ( d ). Mutants were stained with 12.3, 37.0, 111, 333, and 1000, nM Tax and MART/HLA-A2 PE-conjugated streptavidin tetramers. Normalized per cent max mean fluorescence intensity (MFI) is plotted against peptide/HLA-A2 tetramer concentration. This experiment was also performed with pepMHC-Ig dimers with similar results ( Supplementary Fig. 9 ). Full size image Binding studies of soluble RD1 mutants To further examine the binding properties of selected, peptide-specific TCR clones, soluble single-chain TCRs RD1-Tax-1 (identical to A6-X15), RD1-MART1 and RD1-MART1 HIGH were examined for binding to antigen-presenting cell line T2 cells loaded with peptides and/or by surface plasmon resonance (SPR). Binding of soluble RD1-MART1 and RD1-MART1 HIGH to MART1/HLA-A2 complexes on T2 was measured using biotinylated single-chain TCRs. Peptide-loaded T2 cells were incubated with various concentrations of biotinylated TCRs, followed by washing and staining with streptavidin–phycoerythrin (SA–PE). The RD1-MART1 clone yielded positive staining above 500 nM, whereas the RD1-MART1 HIGH TCR yielded positive staining at low nanomolar concentrations, with half-maximum staining at 30 nM ( Fig. 6 ). No staining was observed with Tax/HLA-A2 even at the highest concentration of TCRs. 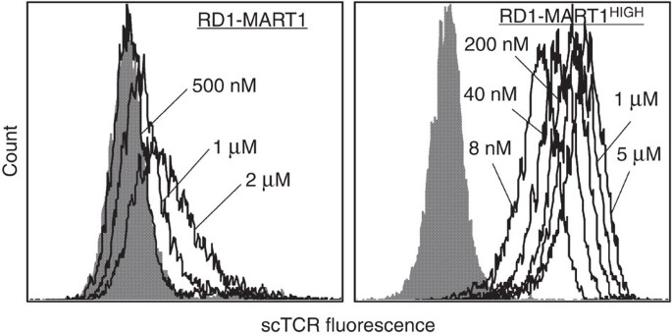Figure 6: Binding of soluble TCRs to antigen-presenting cells. T2 cells were loaded with Tax or MART1, followed by incubation with biotin-labelled RD1-MART1 (left) or RD1-MART1HIGH(right) scTCRs at the indicated concentrations. The shaded grey histograms show staining with Tax-loaded T2 cells at the maximum concentration of TCR for each experiment (2 μM and 5 μM, respectively). Data are representative of two experiments with similar results. Figure 6: Binding of soluble TCRs to antigen-presenting cells. T2 cells were loaded with Tax or MART1, followed by incubation with biotin-labelled RD1-MART1 (left) or RD1-MART1 HIGH (right) scTCRs at the indicated concentrations. The shaded grey histograms show staining with Tax-loaded T2 cells at the maximum concentration of TCR for each experiment (2 μM and 5 μM, respectively). Data are representative of two experiments with similar results. Full size image SPR was performed by flowing scTCR proteins over immobilized pepMHC complexes or flowing pepMHC over immobilized scTCR. Similar to previous studies with the A6-X15 scTCR [34] , the RD1-Tax-1 TCR exhibited a K D value of 84 nM for Tax/HLA-A2 based on equilibrium measurements ( Table 1 ). The first-generation MART1-specific TCR, RD1-MART1, exhibited a K D value of 3.1 μM based on equilibrium measurements. The affinity-matured TCR RD1-MART1 HIGH exhibited a K D value of 68 nM based on kinetic measurements and 247 nM based on equilibrium measurements. An equilibrium titration of RD1-MART1 and RD1-MART1 HIGH with MART1/HLA-A2 or negative controls is shown in Supplementary Fig. 11 . Table 1 Binding properties of RD1 library-derived TCR clones*. Full size table Yeast display, flow cytometry-based titrations with ligands have been used in various studies as a method for examining binding affinities [45] , [46] . The results of SPR studies were consistent with various experiments in which monomers or multimers of the pep/HLA-A2 complexes were used to stain the yeast-displayed forms of these TCRs and half-maximal binding concentrations were determined ( Table 1 ). There was a high degree of specificity of the yeast-displayed scTCR variants for their respective peptides, as even the highest concentrations of the null pepMHC multimers did not bind. Analysis of A6-X15 and RD1-MART1 by MD simulations To gain further insight into the underlying molecular mechanism of peptide specificity, comparative molecular dynamics (MD) simulations were performed on two complexes, A6:Tax/HLA-A2 and RD1-MART1:MART1/HLA-A2. To determine whether MD was a valid method to analyse possible mechanisms of specificity of the RD1 variants, two sets of validation simulations were performed. First, we showed that MD simulations would correctly predict the backbone and side-chain orientations of the CDR3β loop of high-affinity TCR A6-c134 derived from A6 ( Supplementary Methods and Supplementary Fig. 12 ). Second, we determined that MD simulations could accurately predict the insertion of the side chain of residue F100β in the DMF5 TCR (PDB: 3QDG) [6] ( Supplementary Methods and Supplementary Fig. 13 ). For MD simulations of RD1-MART1:MART1/HLA-A2, four different initial models were constructed based on the A6-c134:Tax/HLA-A2 orientation (PDB: 4FTV) as well as three different orientations observed for decameric MART1/HLA-A2 in complex with different MART1-specific TCRs (DMF5, DMF4 and Mel5; PDBs: 3QDG, 3QDM and 3HG1, respectively) [6] , [7] , [47] (see Methods for details). Two distinct peptide–TCR interaction patterns were observed for A6 and RD1-MART1, which could account for their differential peptide-binding specificity and affinity. Key interactions in the A6:Tax/HLA-A2 complex identified by screening for hydrogen bonding and electrostatic interactions included three hydrogen bonds, namely, Y5 Tax -R95β, Y5 Tax -S31α and Y8 Tax -E30β ( Fig. 7a and Supplementary Fig. 14 ). A recent mutational study suggested that A6 interactions with Y8 Tax provided significant binding energy [16] . Consistent with this, the L98β mutations in the present study probably influenced a van der Waals interaction between Y8 Tax and L98β. Our simulations also identified a key hydrogen bond between Y8 Tax and E30β. 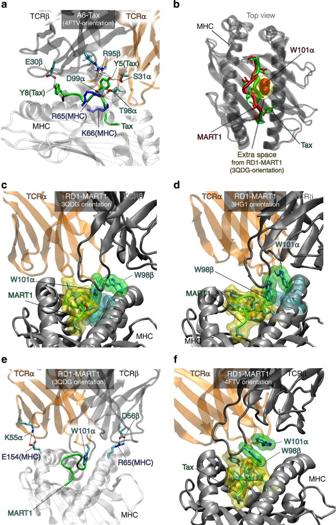Figure 7: MD simulations of RD1 variants. (a) Specific hydrogen bonding and salt-bridge interactions are shown for A6-c134:Tax/HLA-A2. (b) A superposition of A6-c134:Tax/HLA-A2 and RD1-MART1:MART1/HLA-A2 (3QDG/DMF5-orientation), highlighting the extra space created by the curvature of MART1 but not by Tax. (c) Insertion of tryptophan W101α of RD1-MART1 into the interface between MART1 and HLA-A2 in the 3QDG/DMF5 orientation. (d) Insertion of tryptophan W98β of RD1-MART1 into the interface between MART1 and HLA-A2 in the 3HG1/Mel5 orientation. (e) Salt-bridge interactions that occur in the 3QDG/DMF5 orientation of the RD1-MART1:MART1/HLA-A2 complex. (f) The absence of tryptophan insertion in RD1-MART1 when Tax replaces MART1 in the HLA-A2 complex (4FTV/A6-c134 orientation). Figure 7: MD simulations of RD1 variants. ( a ) Specific hydrogen bonding and salt-bridge interactions are shown for A6-c134:Tax/HLA-A2. ( b ) A superposition of A6-c134:Tax/HLA-A2 and RD1-MART1:MART1/HLA-A2 (3QDG/DMF5-orientation), highlighting the extra space created by the curvature of MART1 but not by Tax. ( c ) Insertion of tryptophan W101α of RD1-MART1 into the interface between MART1 and HLA-A2 in the 3QDG/DMF5 orientation. ( d ) Insertion of tryptophan W98β of RD1-MART1 into the interface between MART1 and HLA-A2 in the 3HG1/Mel5 orientation. ( e ) Salt-bridge interactions that occur in the 3QDG/DMF5 orientation of the RD1-MART1:MART1/HLA-A2 complex. ( f ) The absence of tryptophan insertion in RD1-MART1 when Tax replaces MART1 in the HLA-A2 complex (4FTV/A6-c134 orientation). Full size image The MD simulations also identified A6-c134:HLA-A2 interactions involving a salt bridge between D99α and R65 MHC of HLA-A2. In addition, a salt bridge between D99α and K66 MHC of HLA-A2 occasionally formed during the simulations, with the orientation of the D99α side chain being further stabilized by the hydroxyl group of T98α ( Supplementary Fig. 14 ). These contacts probably play a role in further enhancing TCR:HLA-A2 interactions ( Supplementary Fig. 14 ). The importance of T98α and D99α in A6 TCR recognition has recently been established by mutational analysis [16] . Interestingly, the selection of T98α and D99α by Tax/HLA-A2, but not by MART1/HLA-A2 (where K98α and Y99α were selected), also indicates that the peptide has a strong influence on these TCR:HLA-A2 interactions. In contrast to the A6-c134:Tax/HLA-A2 complex, the major stabilizing interaction in RD1-MART1 complexes appeared to be the insertion of a tryptophan side chain from RD1-MART1 (W101α in the 3QDG/DMF5 orientation or W98β in the 3HG1/Mel5 orientation) into the extra space provided by the highly curved topology of the MART1 peptide ( Fig. 7b–d ). This insertion of a tryptophan side chain was not observed in the 4FTV/A6-c134 or 3QDM/DMF4 orientations ( Supplementary Fig. 15 ), a finding also supported by calculations of the solvent accessible surface area ( Supplementary Fig. 16 ). This suggests that the 4FTV/A6-c134 and 3QDM/DMF4 orientations are unlikely to represent optimally bound configurations for the complex, and that the more probable mode of interaction is similar to those observed in the 3QDG/DMF5 or 3HG1/Mel5 crystal structures. The exclusion of a 3QDM/DMF4-like orientation is further consistent with the structural data, as the DMF4 TCR does not use the Vα2 gene segment. The 4FTV/A6-c134 and 3QDM/DMF4 orientations were also characterized by a counter-clockwise rotation (when viewed from the top of the TCR) with regard to the other two orientations. The orientation in 3QDG/DMF5 (but not 3HG1/Mel5) allows the establishment of two salt bridges, K55α with E154 MHC of HLA-A2 and D56β with R65 MHC of HLA-A2, which have interaction probabilities of 51.1% and 97.5%, respectively ( Fig. 7e and Supplementary Fig. 14 ). Thus, although both 3QDG/DMF5 and 3HG1/Mel5 orientations show tryptophan insertion, only the former orientation simultaneously maintains both of these inter-domain salt bridges, making the 3QDG/DMF5 orientation more likely to be representative of the complex ( Fig. 7d,e ). These CDR2 interactions (K55α/E154 MHC and D56β/R65 MHC ) have been described in several TCR complexes [15] , [48] , and they help facilitate the conserved TCR diagonal orientation observed for most TCR:pepMHC complexes [4] , [48] . It is interesting to note that the DMF5:MART1/HLA-A2 structure (PDB: 3QDG), similar to the modelled RD1-MART1:MART1/HLA-A2 complex, also contains the Vα2 region, MART1 and HLA-A2. Although the TCR (DMF5) in the 3QDG/DMF5 structure does not contain a tryptophan in either CDR3, a phenylalanine at position 100 in the CDR3β inserts into the same area as the MART1/HLA-A2 ligand as predicted by the MD simulations ( Supplementary Fig. 17 ). Rosetta sequence tolerance algorithms also showed a strong preference for tyrosine and phenylalanine at position F100β ( Supplementary Fig. 10b ). Although the salt bridges described above are not present, R65 MHC of HLA-A2 plays a key role, as it does in most other complexes [6] , [48] . Finally, we examined what would happen if MART1 were replaced by Tax in the MD simulations of the RD1-MART1:MART1/HLA-A2 complexes. In this simulation, the tryptophan insertion could not be established due to the different backbone topology of the Tax peptide ( Fig. 7f ). In addition, neither of the salt bridges mentioned above formed and the triple hydrogen bonding pattern observed in the A6-Tax/HLA-A2 complex was absent in the MD simulation of the RD1-MART1:Tax/HLA-A2 complex. In addition, when MART1 is replaced by Tax in a model of the complex with A6-c134, A6 was found in the simulation to lose not only the triple hydrogen bonds, but also the D98α-K66 MHC salt bridge. Collectively, these effects probably account for the differential affinity of A6 and RD1-MART1 for MART1/HLA-A2 and Tax/HLA-A2. The results of these MD simulations will require crystal structures to verify. The peripheral T-cell repertoire is shaped by positive and negative selection in the thymus, whereby T cells with TCRs that do not bind to self-pepMHC, or with TCRs that bind too strongly, are deleted [1] , [2] . The wild-type TCRs that have been isolated and characterized biochemically and structurally have been derived from T cells that have made it through these stringent in vivo selection processes. In this study, we created repertoires of TCRs in yeast display libraries that could be selected for pepMHC binding in vitro without the in vivo ‘filters’ that are involved in thymic or peripheral T-cell processes. We believe that this in vitro selection approach can provide additional information about the fundamental basis of pepMHC specificity of TCRs. In addition, the strategy represents a high-throughput system to generate specific TCR leads against the thousands of potential targets represented by viral or cancer peptides, without the need to isolate T-cell clones for each one. Our primary goal in the present study was not to affinity mature a wild-type TCR against its cognate antigen [19] , [20] , [21] , [22] , [23] , [24] , [27] , [28] , [29] , [30] , but to use directed evolution to isolate TCRs with novel specificities against non-cognate antigens. We chose the human TCR A6 as an initial scaffold based on the wealth of information available and previous findings that it is amenable to yeast display and directed evolution [34] . The A6 TCR recognizes at least three distinct HLA-A2-restricted ligands, Tax (LLFGYPVYV), derived from HTLV-1, and two structural mimics of Tax called Tel1p (MLWGYLQYV) and HuD (LGYGFVNYI) [6] , [15] , [49] . Studies of A6 binding to these and various other mutant Tax peptides have shown significant plasticity in CDR3 loops to accommodate a variety of substitutions in the Tax structure [32] , [50] , [51] . Two different libraries of the A6 TCR resulted in TCR variants that bound to the non-cognate antigen MART1/HLA-A2. To the best of our knowledge, this is the first report of ‘switching’ the specificity of a TCR to a completely different peptide by directed evolution. The MART1-specific TCRs from both of the libraries contained similar mutations within the CDR3 loops. In RD1-MART1, a tryptophan (98β) replaced the leucine of the wild-type A6 TCR and mutagenesis showed that the W98β played a key role. In RD2-MART1, a tryptophan at position 101 of the CDR3α was selected and it is possible that it functions in a manner similar to the W98β. In RD1-MART1 a lysine was selected at position 98 of the CDR3α, whereas in RD2-MART1 an arginine was selected at position 102 of CDR3β. Strikingly, the affinity-matured variant of RD1-MART1 (RD1-MART1 HIGH ) evolved four residues in CDR3β (MAGG, 99–102) that were also selected, in a one-amino-acid register shift in the RD2-MART1 clone (MAGG, 98–101). A structure of these mutants will be required to fully understand the underlying molecular basis of MART1 specificity. The two different libraries reported here also yielded higher-affinity TCRs for binding to the Tax/HLA-A2 complex. Here, as with the MART1-specific clones, there was strong selection for specific residues in the CDR3β, including four residues at positions 99–102 (MSAQ), which have been identified previously as yielding a high-affinity phenotype. However, in the context of these residues, there was also strong selective pressure for Tax binding evidenced in the preference for residues in CDR3α. For example, four CDR3α residues within the two different libraries (T98 and D99 in RD1, and S100 and W101 in RD2) were highly restricted in Tax selections and these are the same residues found in the wild-type A6 TCR. This finding supports the idea that both CDR3 loops operate in concert to provide specificity, and higher affinity, for Tax. Interestingly, WT1-specific TCRs were not isolated, despite the presence at position 8 in both Tax and WT1 of a tyrosine that is predicted to be a key residue for binding by A6 (ref. 16 ). The absence of TCR variants that bound WT1 among the A6 libraries again supports the view that multiple regions across the TCR interface are involved in conferring specificity (that is, not only those near the Y8 in these two peptides). It is possible that alternative libraries, with degeneracies in other CDR residues, could yield solutions to WT1 binding. The basis of the specificity switch from Tax to MART1 was also investigated by MD simulations of known structures, or of models of the selected TCRs docked onto structures of these pep/HLA-A2 ligands. MD has previously been used to assess the role of conformational heterogeneity in TCR/pepMHC interactions [50] , [52] . To validate the use of MD simulations to probe functionally relevant TCR:pepMHC interactions, we performed several analyses (see Results), which were in agreement with previously reported results using a variety of biophysical and mutational approaches [15] , [16] . The simulation results indicate that major interactions between the A6 TCR and the Tax/HLA-A2 complex involved Tax residues Y5 and Y8, and HLA-A2 residue R65, along with key TCR residues S31α, T98α, D99α, E30β and L98β. Interestingly, although CDR3α residues T98 and D99 interacted with R65/K66 of HLA-A2 and they were highly conserved in selection with Tax/HLA-A2, this restriction was completely dependent on the peptide. Thus, selection of the RD1 library with MART1 yielded only CDR3α residues K98 and Y99, which must provide very different modes of interaction with the MART1/HLA-A2 complex. The MD simulations of the RD1-MART1 TCR revealed a quite striking mode of interaction that could account for a substantial binding difference between MART1 and Tax complexes. A tryptophan in either CDR3α or CDR3β was inserted into the space created by the curved position of the MART1 backbone, providing significant hydrophobic stabilization. This positioning also oriented the outside of the periphery of the TCR-binding surface, through the two CDR2 loops, to form two salt bridges (one with each HLA-A2 helix). The specificity of RD1-MART1 for MART1 was accounted for in part by the inability of Tax to accommodate this tryptophan conformation and thus to allow optimal orientation and interaction between the TCR and the Tax/HLA-A2 complex. One of the libraries (RD2) yielded TCR variants that were cross-reactive with different pep/HLA-A2 ligands. These cross-reactive clones were selected with either non-cognate ligand, MART1/HLA-A2 or WT1/HLA-A2. The sequences of the cross-reactive clones revealed diversity, but highly restricted residues were selected at particular positions of CDR1α, CDR3α and CDR3β. The consensus sequence of these clones, as represented by clone RD2-WT1, involved the following five residues: I26α, S28α, R100α, S101α and V98β. To gain insight into the basis of the binding of these cross-reactive TCRs and their peptide independence, Rosetta Backrub models were generated for various complexes of this canonical mutant TCR, based on the A6 structure. The wild-type A6:Tax/HLA-A2 structure was compared with the models of the RD2-WT1 TCR in complex with Tax/HLA-A2, MART1/HLA-A2 or WT1/HLA-A2 ( Supplementary Fig. 18a ). None of the five residues in A6 were <3.2 Å from the nearest HLA-A2 residues, although several were involved in contacts with Tax. In striking contrast, all five of the RD2-WT1 residues were predicted to be positioned within 3.2 Å of the HLA helices, including the following paired residues (TCR residue:HLA-A2 residue(s)): I26α:E58, S28α:Y59/W167, R100α:A69/Q72, S101α:R65 and V98β:T73 ( Supplementary Fig. 18b,c ). The highly restricted nature of each of these residues in the cross-reactive TCRs across three different loops suggests that they act in concert to contribute to binding of the HLA-A2 molecule. Importantly, all five residues are predicted to be at a sufficient distance from each peptide to avoid steric clashes that would prevent binding. T cells that expressed TCRs such as these RD2 clones would probably have been negatively selected in the thymus. In fact, relevant to this, transgenic mice containing a single pepMHC as selecting ligand yielded T cells with TCRs that exhibited similar cross-reactive behaviour [53] . In addition, the highly restricted sequences of these TCRs, and those selected with specificity for Tax or MART1, are analogous to the dominance of some TCRs that arise from positive selection on self-peptides in the thymus [2] , [54] . In summary, using a single TCR scaffold we have shown that it is possible to generate novel TCRs against non-cognate pepMHC ligands. To improve the likelihood of isolating specific TCRs de novo against other peptide/HLA-A2 complexes (such as WT1), several approaches can be applied to the design of additional libraries, including the use of a collection of TCR templates with different Vα2 and Vβ regions, degeneracies at other CDR positions and the use of synthetic CDR3 loops with varying amino acid lengths. In addition, it may be possible to start with TCRs such as RD2-WT1 that have a basal affinity for most peptide/HLA-A2 complexes, and to engineer specificity by operating on CDR residues that can provide specific binding energy with peptide residues. Reagents and flow cytometry Antibodies and streptavidin conjugates used to detect yeast surface expression included: anti-HA epitope tag (Clone HA.11; Covance; 1:50), anti-c-myc epitope tag (A21281; Molecular Probes; 1:50), goat anti-mouse IgG F(ab′) 2 AlexaFluor 647 secondary antibody (Molecular Probes; 1:100), goat anti-chicken IgG (H+L) Alexa Fluor 488 and 647 secondary antibodies (Molecular Probes; 1:100) and SA–PE (BD Pharmingen; 1:100). Peptides that bind to HLA-A2 (Tax 11–19 : LLFGYPVYV, MART1 26–35 A27L : ELAGIGILTV, WT1 126–134 : RMFPNAPYL, Survivin 95–104 : LTLGEFLKL, gp100 209–217 : ITDQVPFSV) were synthesized by standard F-moc (N-(9-fluorenyl)methoxycarbonyl) chemistry at the Macromolecular Core Facility at Penn State University College of Medicine (Hershey, PA, USA). In addition, an ultraviolet-cleavable peptide, KILGFVFJV, where J is the photo-labile amino acid residue prepared by standard Fmoc-peptide solid phase synthesis using commercially available Fmoc-3-amino-3-(2-nitro)phenyl propionic acid as a building block, was synthesized at the University of Illinois Protein Sciences Facility as previously described [55] , [56] . HLA-A2 reagents include recombinant soluble dimeric HLA-A2:Ig fusion protein (BD DimerX at indicated concentrations, loaded with 120 M excess peptide) and expressed and refolded HLA-A2 monomers and tetramers. HLA-A2 heavy chain was expressed as inclusion bodies in Escherichia coli and refolded in vitro with an ultraviolet-cleavable HLA-A2 binding peptide and human β-2 microglobulin as described [8] , [55] , [56] , [57] . The HLA-A2 heavy chain contained a biotinylation substrate sequence for in vitro biotinylation (Avidity, BirA enzyme). Peptide exchange with HLA-A2-biotin monomers containing the ultraviolet-cleavable peptide was achieved by exposure to ultraviolet light in the presence of excess peptide (100 × peptide in 1% PBS) [55] , [56] . Monomers were converted to tetramers by incubation at a 4:1 molar ratio of monomer:SA–PE. Staining of yeast cells (10 6 ) was performed on ice for 45–60 min, cells were washed with PBS/BSA (1%) and analysed by flow cytometry with an Accuri C6 flow cytometer. RD1 and RD2 library design Candidate residues for degeneracy were determined by measuring which CDR loop positions would be most likely to allow for contacts with a variety of non-cognate peptides using Rosetta Backrub flexible backbone modelling algorithms ( https://kortemmelab.ucsf.edu/backrub/ ) [58] , [59] . Using the wild-type and high-affinity (c134) A6:Tax/HLA-A2 crystal structures (PDB: 1AO7 and 4FTV, respectively) [8] , [47] as input, Rosetta was used to model HLA-A2-restricted MART1 peptides (MART1 26–35 A27L : ELAGIGILTV, MART1 27–35 : AAGIGILTV 27–35 , MART1 27–35 : ALGIGILTV 27–35 A28L ) and peptides WT1 (RMFPNAPYL), SL9/HIV-gag (SLYNTVATL) and Survivin (LTLGEFLKL) using the Rosetta Multiple Mutation Mutagenesis Module [59] . For modelling purposes, the residue at position ‘0’ of the MART1 26–35 A27L 10-mer peptide was omitted from the prediction. Mutated residues were given a 10-Å radius of effect for the flexible backbone modelling. PyMOL was used to visualize and examine overlays of the lowest energy conformation of each model (The PyMOL Molecular Graphics System, Version 1.5.0.4 Schrödinger, LLC) [60] and CDR loop residues that were within hydrogen boding distance (<3.5 Å) of the MART1 26–35 A27L peptide residues were identified. Based on these models, the frequency of residues within this distance was used to select five residue positions for codon degeneracy (NNS) using the A6-X15 scTCR, which contains stabilizing mutations, as a template [34] . Five codons for this RD1 library (rational design library 1) were chosen, because yeast display libraries can be generated to completely cover this sequence diversity (for example, NNS, 32 5 =3.3 × 10 7 ). Residue numbering is consistent with crystal structures of A6:Tax/HLA-A2 (PDB: 1AO7) [8] and A6-c134:Tax/HLA-A2 (PDB: 4FTV) [47] . A second library (RD2) was based on visual inspection of the A6:Tax (LLFGYPVYV)/HLA-A2 crystal structure, selecting residues that were in close proximity to MART1 (ELAGIGILTV)/HLA-A2 and WT1 (RMFPNAPYL)/HLA-A2 in the overlaid crystal structures. In RD2, five codon positions (TCRα D26, G28, S100 and W101; TCRβ L98) were made degenerate (NNK) with significant variance from the RD1 library. Positions D26α and G28α were chosen primarily due to their proximity (<3.5 Å) to the R1 position of the WT1 peptide in the overlaid structures and the S100α position was chosen due to its proximity (<1 Å) to the N5 position of the WT1 peptide in the overlaid structure. The W101α was varied, as MD data had suggested that this position, if altered, could allow for more loop flexibility. Finally, the L98β was varied, as it participates in a key interaction driving the affinity and specificity of A6 for Tax. Based on results of RD1 library selections, TCRα residue 30 was generated as a binary position (wild-type glutamine or selected threonine), and positions 99–102 in CDR3β were also binary (wild-type A6 residues AAGR or high-affinity A6-X15 MSAQ). Generation and selection of RD yeast display libraries The A6 libraries were expressed in the yeast display plasmid pCT302 (Vβ-L-Vα) [61] , [62] . The RD1 library was synthesized by Genscript (Piscataway, NJ, USA) and the RD2 library by DNA2.0 (Menlo Park, CA, USA) using A6-X15 as a template, that included five framework mutations (S33A, E59D, N62D, N66K and K120I, all in the Vβ domain) and two CDR mutations (A52V and Q106L, both in the Vβ domain) that were isolated previously in a stability screen of the scTCR [34] . The RD1 library also contained four CDR3β mutations (A99M, G100S, G101A and R102Q) that yielded higher affinity binding to Tax/HLA-A2 (ref. 21 ). The sequences of the synthesized genes and additional details of the library construction are provided in Supplementary Methods . The RD1 library was induced in galactose-containing media (SG-CAA) for 48 h, washed with 1 ml 1% PBS/BSA and stained with the following: Tax (LLFGYPVYV), MART1 (ELAGIGILTV) or WT1 (RMFPNAPYL)/HLA-A2-Ig dimers, goat-anti-mouse IgG F(ab′) 2 AlexaFluor 647 secondary antibody (1:100). Cells were washed (1 ml, 1% PBS/BSA) and the most fluorescent cells were selected using a FACS Aria (BD Bioscience). Selection was performed with Tax/HLA-A2-Ig dimer (sort 1: 20 nM, sorts 2–4: 10 nM), MART1/HLA-A2-Ig dimer (sorts 1–2: 500 nM, sorts 3–4: 100 nM, sort 5: 20 nM) and WT1/HLA-A2-Ig dimer (sorts 1–2: 500 nM, sorts 3–4: 100 nM). During the third sort with MART1/HLA-A2 and WT1/HLA-A2 selected, yeast cells were also stained with chicken anti-c-myc antibody (1:50), goat anti-chicken IgY Alexa 488 secondary antibody (1:100) and double positives were isolated to exclude truncated clones. Expression was monitored with anti-HA epitope tag (1:50), goat-anti-mouse IgG F(ab′) 2 AlexaFluor 647 secondary antibody (1:100) and anti-cmyc (1:50), goat-anti-chicken IgG (H+L) AlexaFluor 488 or 647 secondary antibody (1:100). The RD2 library was induced in galactose-containing media (SG-CAA) for 48 h, washed with 25 ml 1% PBS/BSA and stained with 5 μm Tax (LLFGYPVYV) or MART1 (ELAGIGILTV)/HLA-A2 ultraviolet-exchanged HLA-A2 monomers [55] , [56] . Magnetic bead selections were performed using streptavidin MACS microbeads (Miltenyl Biotec), for a total of two selections using MACS LS columns on a QuadroMACS Separator (Miltenyl Biotec). Following two selections, the selected libraries were stained with the following: selecting peptide (Tax, MART1 or WT1)/HLA-A2-Ig dimer and goat-anti-mouse IgG F(ab′) 2 AlexaFluor 647 secondary antibody (1:100). Cells were washed (1 ml, 1% PBS/BSA) and the most fluorescent cells were selected using a FACS Aria (BD Bioscience) high-speed sorter. Selections were performed with 1 nM and 100 nM peptide/HLA-A2 for selecting cognate antigen Tax and non-cognate antigen MART1 (ELAGIGILTV), respectively. Expression was monitored with anti-HA epitope tag (1:50), followed by goat-anti-mouse IgG F(ab′) 2 AlexaFluor 647 secondary antibody (1:100) or anti-cmyc (1:50) followed by goat-anti-chicken IgG (H+L) AlexaFluor 647 secondary antibody (1:100). Generation and selection of RD-MART1 yeast display libraries CDR3 libraries were generated by splicing by overlap extension PCR spanning five adjacent codons at a time (two libraries in the CDR3β loop spanning residues 97–101 and 99–103; one library in the CDR3α loop spanning residues 98–102) [63] using the RD1-MART1 scTCR clone selected from the RD1 library as a template. Details of the libraries are described in Supplementary Methods . The combined library was induced in galactose-containing media (SG-CAA) for 48 h, washed with 1 ml 1% PBS/BSA and stained with MART1 (ELAGIGILTV)/HLA-A2-Ig dimer goat-anti-mouse IgG F(ab′) 2 AlexaFluor 647 secondary antibody (1:100). Cells were washed (1 ml, 1% PBS/BSA) and the most fluorescent cells were selected using a FACS Aria (BD Bioscience) high-speed sorter. Selection was performed with MART1 (ELAGIGILTV)/HLA-A2-Ig dimer (sort 1: 200 nM, sort 2: 1 nM). Expression was monitored with anti-HA epitope tag (1:50), followed by goat-anti-mouse IgG F(ab′) 2 AlexaFluor 647 secondary antibody (1:100) or anti-cmyc (1:50) followed by goat-anti-chicken IgG (H+L) AlexaFluor 647 secondary antibody (1:100). Isolation and staining of high-affinity clones Following sorting with various selecting antigen, library colonies were isolated by plating limiting dilutions. Colonies were expanded and induced in galactose-containing media (SG-CAA) for 48 h, washed with 1 ml 1% PBS/BSA and stained with various concentrations of peptide/HLA-A2-Ig dimer goat-anti-mouse IgG F(ab′) 2 AlexaFluor 647 secondary antibody (1:100) or various concentrations of ultraviolet-exchanged peptide/HLA-A2 monomers [55] , [56] SA–PE (1:100). Cells were washed (1 ml, 1% PBS/BSA) and analysed on an Accuri C6 flow cytometer. Plasmids were recovered using Zymoprep Yeast Plasmid Miniprep II (Zymo Research) and introduced back into E. coli via heat-shock transformation into Subcloning Efficiency DH5α Competent Cells (Invitrogen). E. coli cells were expanded and plasmids were isolated using QIAprep Spin Miniprep Kit (Qiagen, Valencia, CA). Sequences of individual clones were determined by Sanger sequencing. Expression and purification of soluble scTCR fragments RD1-MART1 and RD1-MART1 HIGH were introduced into the pET28a expression vector with a C-terminal AviTag (Avidity) using Nco I and Eco RI restriction sites (forward primer: 5′—TAT ACC ATG GGC AGC AGC CAT CAT CAT CAT CAT CAC AGC AGC GGC CTG GTG CCG CGC GGC AGC AAT GCT GGT GTA ACA CAA ACG CC—3′, reverse primer: 5′—T TTA GAA TTC TTA TTC GTG CCA TTC GAT TTT CTG AGC CTC GAA GAT GTC GTT CAG ACC GCC ACC GTC TGG AGT GAC CAC AAC CTG GGT—3′. Plasmids were transformed into the BL21-DE3 cell line (NEB), expanded and induced for expression. Following induction, cells were passed through a microfluidizer (Microfluidics Corporation, Newton, MA, USA), inclusion bodies were isolated and protein was purified as previously described [64] . Soluble scTCR were refolded and purified with Ni-NTA agarose resin (Qiagen) followed by gel filtration (Superdex 200, GE Healthcare). Folded scTCRs were biotinylated in vitro (Avidity, BirA enzyme). Biotinylation was verified by gel shift with streptavidin by SDS–PAGE. Surface plasmon resonance The binding of purified refolded scTCR proteins to cognate peptide/HLA-A2 was monitored with SPR using a Biacore 3000 instrument. Kinetic and equilibrium binding data were determined by immobilizing biotinylated pepMHC monomers on a neutravidin-coated CM5 sensor chip to 400–800 response units. A null pepMHC molecule was immobilized to the reference cell. Purified soluble scTCRs were diluted to various concentrations in Biacore buffer (10 mM HEPES, 150 mM NaCl, 3 mM EDTA, 0.005% Tween-20, pH 7.4) and flowed over the reference and experimental flow cells at 30 μl min −1 at 25 °C. Binding of the scTCR to the null complex was subtracted from the scTCR binding to the experimental complex, to correct for bulk shift and any nonspecific binding. In addition, data obtained from injections with no analyte were subtracted from each concentration. Curve fitting and determination of on-rates, off-rates and kinetic-based K D measurements were performed using BIAEvaluation 4.1.1 software. Equilibrium K D values were determined by calculating half-max values from non-linear regression analysis of plots of the maximum response units for each scTCR concentration. For equilibrium SPR values in this orientation, n =3 for RD1-MART1 and n =2 for RD1-MART1 HIGH . For kinetic SPR values in this orientation, n =1 for A6-X15 and RD1-MART1 HIGH . In addition, an independent SPR experiment was performed in the reverse orientation (that is, scTCR immobilized) to facilitate the use of multiple control pepMHC analytes. For this experiment, steady-state binding was measured as previously described [65] . Experiments were performed at 25 °C with solution conditions of 10 mM HEPES, 3 mM EDTA, 150 mM NaCl, 0.005% surfactant P20, pH 7.4. RD-MART1 and RD-MART1 HIGH were coupled to the surface of a CM5 sensor chip via amine linkage to a density of ~1,000 response units. Soluble MART1/HLA-A2, Tax/HLA-A2 and gp100/HLA-A2 were injected over the surface in a series of concentration points until steady state was attained. Each pepMHC concentration series was injected twice. Data was processed in BiaEvaluation 4.1 and globally analysed in Origin 7.5. Values from repeated experiments in both orientations were averaged and reported with s.d. Binding of TCRs to peptide-pulsed antigen-presenting cells HLA-A2 + human cell line T2 was incubated at 37 °C for 2–3 h with 1 μM MART1 (ELAGIGILTV) or Tax (LLFGYPVYV) peptide. Cells were washed with 1% PBS/BSA and incubated on ice for 1 h with biotinylated scTCR at various concentrations. Cells were washed with 1% PBS/BSA followed by incubation with SA–PE (1:100) for 30–45 min on ice. Cells were washed twice and analysed using an Accuri C6 Flow Cytometer. Site-directed mutagenesis of TCRs Site-directed mutants at position 98 of TCRβ A6-X15, L98W and L98M; RD1-MART1 W98L; RD1-MART1 HIGH W98L; and RD2-MART1 M98L were made using a QuikChange II Site-Directed Mutagenesis Kit (Agilent Technologies). Yeast cells displaying the single-site mutants were titrated with cognate-peptide-exchanged HLA-A2 SA–PE tetramers at 12.3, 37.0, 111, 333, and 1000, nM, and analysed by flow cytometry. Values were normalized using nonlinear regression analysis. Changes in binding affinity were approximated by determining the scTCR concentrations at one-half maximal wild-type binding. Independent experiments were performed with peptide/HLA-A2-Ig dimers with similar results ( Supplementary Fig. 9 ). MDs simulations of A6 and modelled RD1-MART1 Four molecular complexes were modelled and simulated: A6:Tax/HLA-A2, A6:MART1/HLA-A2, RD1-MART1:Tax/HLA-A2 and RD1-MART1:MART1/HLA-A2. For A6:Tax/HLA-A2, the crystal structure of the high-affinity (c134) A6:Tax/HLA-A2 crystal structure (PDB: 4FTV) [47] was used to construct the initial model for the simulation. The same crystal structure was also used as the template to model the RD1-MART1:MART1/HLA-A2 complex, as no experimentally derived structure is currently available for this complex. However, given the presence of MART1/HLA-A2 in other crystal structures showing variable orientations between the TCR and MHC components (TCRs DMF5 (PDB: 3QDG) [6] , DMF4 (PDB: 3QDM) [6] and Mel5 (PDB: 3HG1) [7] ), four different orientations have been also modelled and simulated to investigate the complexes that included MART1 (see Supplementary Methods ). These systems are referred to as the 4FTV/A6-c134, 3QDG/DMF5, 3QDM/DMF4 and 3HG1/Mel5 orientations, respectively. After the initial equilibration phase, each system was subjected to production runs: 100 ns for groups involving the A6-c134 TCR in 4FTV|3QDG/DMF5 conformations, 170 ns for all RD1-MART1 TCR orientations and 50 ns for groups involving A6-c134 TCR in 3HG1/Mel5|3QDM/DMF4 conformations. How to cite this article: Smith, S. N. et al. Changing the peptide specificity of a human T-cell receptor by directed evolution. Nat. Commun. 5:5223 doi: 10.1038/ncomms6223 (2014).